Unusual double ligand holes as catalytic active sites in LiNiO2 Designing efficient catalyst for the oxygen evolution reaction (OER) is of importance for energy conversion devices. The anionic redox allows formation of O-O bonds and offers higher OER activity than the conventional metal sites. Here, we successfully prepare LiNiO 2 with a dominant 3 d 8 L configuration ( L is a hole at O 2 p ) under high oxygen pressure, and achieve a double ligand holes 3 d 8 L 2 under OER since one electron removal occurs at O 2 p orbitals for Ni III oxides. LiNiO 2 exhibits super-efficient OER activity among LiMO 2 , R MO 3 (M = transition metal, R = rare earth) and other unary 3d catalysts. Multiple in situ/operando spectroscopies reveal Ni III →Ni IV transition together with Li-removal during OER. Our theory indicates that Ni IV (3 d 8 L 2 ) leads to direct O-O coupling between lattice oxygen and *O intermediates accelerating the OER activity. These findings highlight a new way to design the lattice oxygen redox with enough ligand holes created in OER process. The electrocatalysis of the oxygen evolution reaction (OER) is at the core of many energy conversion devices, such as water and CO 2 electrolysers, and metal-air batteries [1] , [2] , [3] . Because of the sluggish kinetics of OER, the exploration of OER electrocatalysts with high intrinsic activity plays a decisive role in determining the device performance, and thus the fundamental understanding of OER mechanisms is essential [4] , [5] , [6] , [7] . The conventional adsorbate evolution mechanism, involving multiple adsorbed intermediates with highly correlated adsorption strengths, exhibits a minimum theoretical overpotential of about 0.37 V [8] , [9] . This limitation has been circumvented by a recently identified mechanism [10] , [11] —the lattice oxygen oxidation mechanism—wherein the oxygen ligands are electrochemically activated, coupled directly with *O intermediates, and released from the lattice matrix [4] . Lattice-oxygen-activated electrocatalysts, such as 3 d late-transition-metal (TM) oxides with high metal oxidation states, universally feature a high TM-O covalency with a strong orbital hybridization between TM 3 d and O 2 p orbitals, which enables intramolecular electron transfer from the oxygen ligands to the TM cations, leaving ligand holes for lattice oxygen activation [4] , [10] . Such an anionic redox mechanism is well documented in lithium-ion-battery (LIB) cathodes [12] and thermal oxidative catalysis [13] . Ni III oxides are intrinsically anionic-redox-active. Here we use the notation Ni III rather than Ni 3+ as a reminder that the formally trivalent Ni ion is in a highly covalent situation where holes in the oxygen 2 p ligands play a significant role. Ni III oxides such as R NiO 3 , R SrNiO 4 ( R = rare earth element), and LiNiO 2 are in the negative charge-transfer energy regime (Δ < 0, Fig. 1a ), leading to 3 d 8 L ( L denotes a ligand hole located on a molecular orbital formed by the O 2 p orbitals) as the dominant ground state configuration, instead of the conventional 3 d 7 (Δ > 0, Fig. 1b ) [14] , [15] , [16] , [17] , [18] , [19] . It is well known that as the Ni III oxidized to Ni IV , the electron removal in such charge transfer system should happen in the O 2 p band rather than the Ni 3 d band [20] , resulting in a 3 d 8 L 2 configuration, namely double O 2 p hole states (Fig. 1a ). Fig. 1: Schematic single-electron removal spectra of Ni III oxides with a formal 3 d 7 filling. a Δ < 0 and b Δ > 0 scenarios. Charge-transfer energy Δ : energy cost for electron transferring from the O 2 p band to the Ni 3 d band, and U : energy cost for electron transferring from the occupied 3 d band to the unoccupie d 3 d band. The hybridization between Ni 3 d and O 2 p is neglecte d for sim p licity. The Fermi level (E F ) is shown as a vertical dash black line and the O 2 p band is used as the energy reference considering the position of E F is arbitrary in the band gap. Full size image Based on the lattice oxygen oxidation mechanism, we proposed that a catalyst featuring double ligand hole states would endow high OER activity. To test our prediction, LiNiO 2 is employed as the precatalyst for the double ligand hole states considering that it has an edge-shared Ni-O-Ni network, which is more stable than the corner-shared network in R NiO 3 [21] and R SrNiO 4 [22] . In addition, as a well-known cathode material of LIB, LiNiO 2 can be easily delithiated and oxidized to form Ni IV ions [23] , [24] , although this oxidizing process is rarely observed during OER in aqueous electrolytes. The stabilization of the highly active Ni IV has been recently attributed to the high-entropy charge-glass-like state of LiNiO 2 [17] . The electronic structure of LiNiO 2 is found to have many nearly degenerate states composed of [NiO 6 ] octahedra with 3 d 8 , 3 d 8 L and 3 d 8 L 2 configurations [17] . The LiNiO 2 system can fluctuate between these states such that the hole states on the oxygen ligands are stabilized by the entropy term of the free energy. In this study, a pristine Ni 2+ -free LiNiO 2 sample was prepared using high-pressure O 2 , and its structure was comprehensively characterized using multiple complementary techniques, including microscopic techniques, X-ray diffraction (XRD), and X-ray absorption spectroscopy (XAS) at the Ni K , Ni L 3,2 , and O K edges. The electrocatalytic properties of LiNiO 2 was robustly assessed using rotating ring disk electrodes (RRDE). The delithiation, oxidation and resulting structural transition of LiNiO 2 during OER were probed using operando XRD, XAS and Raman spectroscopies. Combined analysis of the operando results, density function theory (DFT) calculation and in situ differential electrochemical mass spectrometry (DEMS) reveals that the enhanced OER activity of LiNiO 2 is originated from the structurally stabilized Ni IV with a 3 d 8 L 2 configuration. Structural characterization of LiNiO 2 The crystalline phase and morphology of the as-prepared LiNiO 2 were characterized using synchrotron X-ray diffraction (XRD) and transmission electron microscopy (TEM) (Fig. 2 ). The XRD pattern of LiNiO 2 is well-matched with the standard pattern of R-3m LiNiO 2 (JCPDS No. 09-0063) without any noticeable crystalline impurities (Fig. 2a and Supplementary Fig. 1 ). The sharp diffraction peaks, and the well separation of (006) and (10-2) and of (10-8) and (110), indicate a well-crystalized layered structure with a low degree of Li + /Ni 2+ intermixing (Supplementary Fig. 1 ) [23] , [25] . Rietveld refinement was carried out to obtain the crystal structural parameters of the as-prepared LiNiO 2 (Fig. 2a ), yielding a good fit for the R-3m structure and ~3.9% Ni occupancy in the [LiO 2 ] layers, demonstrating the high-purity of the sample. The single crystalline nature of the as-prepared LiNiO 2 is suggested by TEM techniques (Fig. 2b–d ). A typical selected-area electron diffraction (SAED) pattern of LiNiO 2 shows clear diffraction spots that can be indexed to the R-3m structure of LiNiO 2 along the [010] zone axis (Fig. 2b ). High-resolution TEM (HRTEM) images of the thin parts of LiNiO 2 display uniform lattice fringes of (003) and (104) of the R-3m structure, respectively (Fig. 2c and Supplementary Fig. 2 ). Aberration-corrected high-angle annular dark-field scanning transmission electron microscopy (HAADF-STEM) images were also recorded to directly visualize the Ni atomic arrangement along the edges, which well matches the (003) lattice plane of R-3m LiNiO 2 (Fig. 2d ). TEM, scanning electron microscopy (SEM) and atomic force microscopy (AFM) suggest that the general morphology of the as-prepared LiNiO 2 is nanoflakes with 200 − 400 nm in the lateral size and ~10 nm in the layer thickness (Supplementary Fig. 3 and Fig. 2e ). LiNiO 2 -raw, a LiNiO 2 sample prepared without the second annealing step under high-pressure O 2 , shares a similar morphology with the LiNiO 2 (Supplementary Fig. 4 ). Fig. 2: Structural characterization of the as-prepared LiNiO 2 . 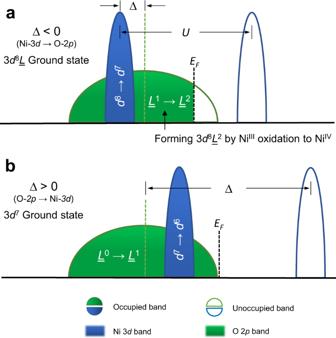Fig. 1: Schematic single-electron removal spectra of NiIIIoxides with a formal 3d7filling. aΔ< 0 andbΔ> 0 scenarios. Charge-transfer energyΔ: energy cost for electron transferring from the O 2pband to the Ni 3dband, andU: energy cost for electron transferring from the occupied 3dband to the unoccupied3dband. The hybridization between Ni 3dand O 2pis neglectedfor simplicity. The Fermi level (EF) is shown as a vertical dash black line and the O 2pband is used as the energy reference considering the position of EFis arbitrary in the band gap. a A synchrotron XRD pattern (18 keV incident beam energy, λ = ~0.6888 Å) and a Rietveld refinement fit with the refined structural parameters listed in Supplementary Table 1 , along with the structural model of R-3m LiNiO 2 which consists of alternate [LiO 2 ] and [NiO 2 ] layers formed by edge-sharing [LiO 6 ] or [NiO 6 ] units. A set of extra diffraction peaks are from graphitic carbon of carbon paper and two broad diffraction peaks at 12° and 18° are from the sample holder. b A typical SAED pattern of LiNiO 2 along a [010] zone axis of the R-3m structure, c a HRTEM image and its fast Fourier transform pattern, showing the (003) lattice fringes, and d an AC-HAADF-STEM image projected perpendicular to the (003) lattice plane. e An AFM image and the corresponding thickness profile across the horizontal red line. Full size image The local coordination environment of transition metal ions can be obtained by extended X-ray absorption fine structure (EXAFS) spectra at the corresponding K edges [26] , [27] . The Ni local coordination of LiNiO 2 resemble that of NiO and Ni(OH) 2 , with two dominant peaks at ~1.8 and ~2.8 Å, which are attributed to Ni–O and Ni–Ni scattering paths within and between the edge-sharing [NiO 6 ] units, respectively (Fig. 3a and Supplementary Fig. 5 ). For these peaks, LiNiO 2 shows a shorter radial distance than those of Ni(OH) 2 and NiO, supporting the presence of a shorter Ni-O bond length due to the higher formal oxidation state of Ni. Fig. 3: XAS characterisation of the as-prepared LiNiO 2 . a Fourier transforms of k 3 -weigted EXAFS spectra of LiNiO 2 , LiCoO 2 (R-3m) and NiO, and b XANES spectra of LiNiO 2 and Ni references (NiO, Ni(OH) 2 , and KNiIO 6 ) at the Ni K edge. The amplitude of LiNiO 2 EXAFS spectra is adjusted for a clear comparison, and the Fourier transforms were phase-corrected. TEY-XAS spectra of LiNiO 2 c at the Ni L 3 edge and d at the O K edge, along with NiO and γ-NiOOH as the Ni and O references. Full size image From an ionic picture, low spin Ni III ions adopt a ( t 2 g ) 6 ( e g ) 1 configuration in an octahedral crystal field and are Jahn-Teller (JT)-active, so that one can expect a strong local distortion of the [NiO 6 ] octahedra to remove the degeneracy of the e g orbitals. There are local distortions of the [Ni III O 6 ] units here, as evidenced by the broader first coordination shell at 1.7 A and a larger disorder factor (σ 2 ) of LiNiO 2 by fitting R -space EXAFS spectra, as compared with that of the analogous R-3m LiCoO 2 (Co III , ( t 2 g ) 6 ( e g ) 0 , Fig. 3a , Supplementary Fig. 6 , and Table 1 ). Two distortion mechanisms are proposed. One is the conventional local JT distortion, as suggested by previous EXAFS studies of LiNiO 2 [28] , [29] , with four short Ni-O (~1.920 Å) and two long Ni-O (~2.069 Å) bonds in the [Ni III O 6 ] octahedra (Table 1 and Supplementary Fig. 7a ). However, pure JT distortion fails to explain the neutron-pair distribution function and electronic structure of LiNiO 2 ; therefore, a [NiO 6 ]-size disproportionation (SD) mechanism was proposed, where the number of Ni−O short and Ni−O long is equal [17] (Table 1 and Supplementary Fig. 7b ). Based on these two possible structural models, EXAFS fitting using two Ni−O coordination shells was performed. Both models gave comparable but better fits of the EXAFS data than that using only one Ni–O scattering path (Table 1 and Supplementary Fig. 7c ), supporting the presence of distorted [Ni III O 6 ] in pristine LiNiO 2 . To distinguish JT distortion from SD, double cluster simulation would be needed to simulate the Ni- L 2,3 XAS spectrum of LiNiO 2 [16] , which is beyond the scope of this study. Table 1 Structural parameters of LiNiO 2 , LiCoO 2 , and NiO, obtained from EXAFS fitting a Full size table The oxidation state of the as-prepared LiNiO 2 was assessed by X-ray absorption near edge structure (XANES) spectroscopy (Fig. 3b ). At the Ni K edge, the energy position of LiNiO 2 locates in-between those of Ni 2+ (NiO and Ni(OH) 2 ) and Ni IV references (KNiIO 6 ), suggesting that the Ni of the LiNiO 2 is in the intermediate oxidation state between Ni 2+ and Ni IV . Assuming that the formal oxidation state of Ni is proportional to the energy at 0.7 edge jump height, the average Ni oxidation state of LiNiO 2 can be quantified as ~3.0 (Supplementary Fig. 9 ), in a good agreement with the nominal value. The detailed electronic structure at the surface region can be obtained by total electron yield soft X-ray absorption spectra (TEY-sXAS) at the L 3 edges. The multiplet spectral feature and the energy position at the L 3 edges of 3 d elements are highly sensitive valence state and local environments [30] , [31] , [32] , [33] . Figure 3c shows the Ni L 3 edge sXAS of LiNiO 2 , along with those of NiO and γ-NiOOH as the Ni 2+ and Ni III references, respectively. 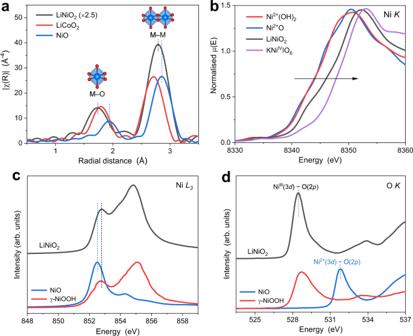Fig. 3: XAS characterisation of the as-prepared LiNiO2. aFourier transforms ofk3-weigted EXAFS spectra of LiNiO2, LiCoO2(R-3m) and NiO, andbXANES spectra of LiNiO2and Ni references (NiO, Ni(OH)2, and KNiIO6) at the NiKedge. The amplitude of LiNiO2EXAFS spectra is adjusted for a clear comparison, and the Fourier transforms were phase-corrected. TEY-XAS spectra of LiNiO2cat the NiL3edge anddat the OKedge, along with NiO and γ-NiOOH as the Ni and O references. Both the multiplet spectral features and energy positions of the Ni- L 3 edge are very similar to those of γ- NiOOH, indicating that the Ni of LiNiO 2 is in the formal +3 oxidation state. The dominant peak for both γ-NiOOH and LiNiO 2 locates at ~855 eV, much higher than that of NiO at ~853 eV, and further inspection reveals that the low-energy peak of LiNiO 2 locates ~0.3 eV higher than the dominant peak of NiO in Fig. 3c . The low-energy peak is an intrinsic spectral feature of Ni III as found in theoretical and experimental XAS [15] , [16] and high-quality single crystal LaNiO 3 and NdSrNiO 4 [21] , [22] In addition, Ni III (3 d 8 L ) in our LiNiO 2 is supported by theoretical simulation of the Ni L 3,2 XAS in Supplementary Fig. 10a , where the LiNiO 2 spectra can be nicely reproduced by the full multiplet cluster calculation with a nominal 3 d 8 L configuration. Our LiNiO 2 is free from Ni 2+ impurity that often observed in the literature (Supplementary Fig. 10b ). The Ni valence state and Ni-O covalency were further studied by the O -K sXAS. The pre-edge peak below 533 eV can be assigned to the unoccupied 3 d e g hybridised with O 2 p orbitals. An increase in the valence state of the 3 d element correlates with a shift of the pre-edge to lower energy and an enhancement of the spectral intensity due to the strong covalence [21] , [34] , [35] . The O- K sXAS of LiNiO 2 is dominated by a strong peak at 528.2 eV without obvious contribution of a peak at 531.9 eV found from NiO (Fig. 3d ). Thus, TEY-sXAS at both the Ni L 3 edges and the O K edge suggest that the surface Ni oxidation state of LiNiO 2 is Ni III and free from Ni 2+ impurities. Electrochemical measurements The OER activity of LiNiO 2 was studied using rotating ring disk electrodes (RRDE, disk: glassy carbon, ring: Pt) at 1600 rpm. The potential of the Pt ring was held at 0.42 V throughout the measurements, so that O 2 once generated on the disk can be collected and electrochemically reduced on the ring (Fig. 4a and Supplementary Fig. 11 ), which enables the determination of OER onset potentials. The OER activity of LiNiO 2 was estimated using linear sweep voltammetry (LSV) in Ar-saturated and Fe-free 1 M KOH and compared with the benchmark IrO 2 (99.9%) catalyst and a NiOOH reference. The LiNiO 2 shows the best OER geometric activity (Fig. 4b , current density normalized by disk electrode area) and intrinsic activity (Supplementary Fig. 13 , current density normalized by electrochemical surface area), with the potential to achieve 10 mA cm geo −2 (E@10 mA cm geo −2 , ~1.545 V) lower than those of IrO 2 (~1.558 V) and NiOOH (~1.753 V). In addition, LiNiO 2 shares a Tafel slope (53 mV dec −1 ) similar to IrO 2 (54 mV dec −1 ) and distinguishes itself from conventional NiOOH (96 mV dec −1 , Fig. 4c ), indicating rapid OER kinetics of LiNiO 2 . Compared to the reported overpotential values of LiMO 2 (M = Co and Fe), and R MO 3 ( R = Rare earth elements, M = Fe, Co and Ni) and other unary 3 d transition metal catalysts, our LiNiO 2 requires much less overpotential to achieve certain current density (Fig. 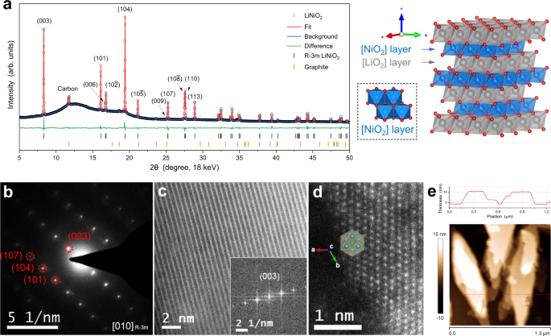4d ), demonstrating the unique electrochemical properties to facilitate OER. Fig. 2: Structural characterization of the as-prepared LiNiO2. aA synchrotron XRD pattern (18 keV incident beam energy, λ = ~0.6888 Å) and a Rietveld refinement fit with the refined structural parameters listed in Supplementary Table1, along with the structural model of R-3m LiNiO2which consists of alternate [LiO2] and [NiO2] layers formed by edge-sharing [LiO6] or [NiO6] units. A set of extra diffraction peaks are from graphitic carbon of carbon paper and two broad diffraction peaks at 12° and 18° are from the sample holder.bA typical SAED pattern of LiNiO2along a [010] zone axis of the R-3m structure,ca HRTEM image and its fast Fourier transform pattern, showing the (003) lattice fringes, anddan AC-HAADF-STEM image projected perpendicular to the (003) lattice plane.eAn AFM image and the corresponding thickness profile across the horizontal red line. Amongst the previously reported LiNiO 2 and even Fe-doped LiNiO 2 , the as-prepared sample exhibit superior E@10 mA cm −2 and Tafel slopes, highlighting the excellent activity of pristine LiNiO 2 (Supplementary Table 2 ). Fig. 4: Electrochemical measurements and surface chemistry of LiNiO 2 . a Schematic illustration of a rotating ring disk electrode (RRDE, ring: Pt, disk: glassy carbon). b Linear sweep voltammograms and c Tafel plots of LiNiO 2 , NiO-derived NiOOH, IrO 2 (99.9% metal basis, Adamas-beta) and carbon (Vulcan XC-72R) in Ar-saturated 1 M KOH solution, along with the corresponding Pt ring current shown in the inset (the onset potential of OER indicated by arrows). d OER activity comparison of the as-prepared LiNiO 2 to LiMO 2 (M = Co and Fe), and R MO 3 ( R = Rare earth elements, M = Fe, Co and Ni) and other unary 3d transition metal catalysts (Supplementary Table 3 ). e Stability test of LiNiO 2 in 1 M KOH at 10 mA cm −2 (on carbon paper) and (the inset of e ) linear sweep voltammograms of LiNiO 2 before and after the stability test. f Window-opening cyclic voltammograms of LiNiO 2 in Fe-free 1 M KOH with stepwise decreasing the lower potential limits, showing the evolution of redox peaks (magnified in the corresponding insets) and the deterioration of OER current. The voltammograms were collected under 1600 rpm with a sweep rate of 5 mV s −1 , and IR drops of the voltammograms were determined by EIS prior to the measurements and compensated. g Operando Raman spectra of LiNiO 2 at 1.56 V with and without being cycled through Ni 2+ /Ni III redox. Full size image The stoichiometric structure of LiNiO 2 is essential to achieve high OER activity. LiNiO 2 -raw was also characterized and compared with the pristine LiNiO 2 , as the high-pressure or high-flow-rate O 2 during synthesis has been found to be essential for stabilizing Ni III and minimizing oxygen vacancies in LiNiO 2 and LiNiO 2 -based cathode materials [36] , [37] . The LiNiO 2 -raw shares similar morphology with the LiNiO 2 (Supplementary Fig. 4 ) but has ~4.6% oxygen vacancies ( vs . ~0.4% in LiNiO 2 ) as characterized by XRD refinement (Supplementary Fig. 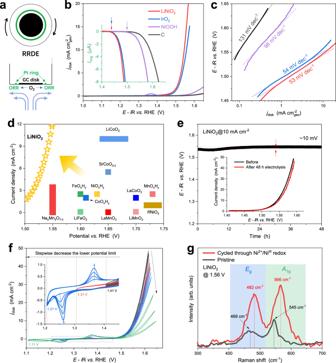Fig. 4: Electrochemical measurements and surface chemistry of LiNiO2. aSchematic illustration of a rotating ring disk electrode (RRDE, ring: Pt, disk: glassy carbon).bLinear sweep voltammograms andcTafel plots of LiNiO2, NiO-derived NiOOH, IrO2(99.9% metal basis, Adamas-beta) and carbon (Vulcan XC-72R) in Ar-saturated 1 M KOH solution, along with the corresponding Pt ring current shown in the inset (the onset potential of OER indicated by arrows).dOER activity comparison of the as-prepared LiNiO2to LiMO2(M = Co and Fe), andRMO3(R= Rare earth elements, M = Fe, Co and Ni) and other unary 3d transition metal catalysts (Supplementary Table3).eStability test of LiNiO2in 1 M KOH at 10 mA cm−2(on carbon paper) and (the inset ofe) linear sweep voltammograms of LiNiO2before and after the stability test.fWindow-opening cyclic voltammograms of LiNiO2in Fe-free 1 M KOH with stepwise decreasing the lower potential limits, showing the evolution of redox peaks (magnified in the corresponding insets) and the deterioration of OER current. The voltammograms were collected under 1600 rpm with a sweep rate of 5 mV s−1, and IR drops of the voltammograms were determined by EIS prior to the measurements and compensated.gOperando Raman spectra of LiNiO2at 1.56 V with and without being cycled through Ni2+/NiIIIredox. 14 and Supplementary Table 4 ), and a significant fraction of Ni 2+ impurities as shown in Ni- K XAS (Supplementary Fig. 15 ) and surface sensitive TEY-sXAS at the Ni L 3 and O K edges (Supplementary Fig. 16 and 17 ). We found that the off-stoichiometric structure of LiNiO 2 -raw yields reduced OER activity (Supplementary Fig. 18 ). From the ring current of the RRDE, the OER onset potentials of LiNiO 2 , IrO 2 and NiOOH were estimated as ~1.437, ~1.438 and ~1.495 V, respectively (Fig. 4b and Supplementary Fig. 11 ), indicating that LiNiO 2 activates the oxidation of water at a much lower overpotential than NiOOH. The OER activity of NiOOH is consistent with a common understanding that Ni (oxy)hydroxides without Fe doping and without the presence of Fe in the electrolyte are poor OER electrocatalysts [38] , [39] , [40] . Thus, from perspectives of overpotentials, Tafel slopes and onset potentials, the electrocatalytic properties of LiNiO 2 for OER is as good as the state-of-the-art IrO 2 and outperforms the standard NiOOH. The stability of LiNiO 2 was measured using chronopotentiometry at 10 mA cm −2 (Fig. 4e ). LiNiO 2 largely maintained its initial potential, which gradually increased by ~10 mV for the first 18 h, and then remained constant for the subsequent 30 h. The high stability of LiNiO 2 is also indicated by the little activity deterioration in LSV before and after the 48 h stability test (the inset of Fig. 4e ). One may be interested in the stability of LiNiO 2 as an OER electrocatalyst, as LiNiO 2 is known to suffer from severe capacity degradation as a cathode material for LIB. The fast capacity fading is generally observed in high voltage region >4.1 V vs . Li + /Li, resulting from a large content of delithiation in Li x NiO 2 (x < 0.3) and in turn structural collapse [23] , [41] , [42] . If the highest cut-off voltage would be limited to 4.1 V vs . Li + /Li, the capacity of LiNiO 2 could retain >95% of its initial capacity after >100 cycles [41] , [43] . However, operation potentials for our OER are below 1.8 V vs . RHE which corresponds to only 4.03 V vs . Li + /Li in battery operation. The interconversion of Ni 2+ -based (hydr)oxides to NiOOH is usually indicated by Ni 2+ /Ni III redox peaks in the potential window of 1.2–1.4 V ( vs . RHE); therefore, the formation of NiOOH from LiNiO 2 was investigated using window-opening cyclic voltammetry. As shown in Fig. 4f , the lower potential limit decreased stepwise from 1.41 V (used in Figs. 4a ) to 1.11 V, close to the values generally used in previous studies [44] , [45] , [46] , [47] , [48] , [49] . When the lower potential limit was set to 1.41 V, the OER current is optimal and remains stable over multiple CV cycles. However, decreasing the limit to ~1.21 and ~1.11 V deteriorates the OER current significantly, accompanied by the appearance and gradual increase of redox peaks at ~1.36 (anodic) and ~1.26 V (cathodic), indicating the formation of redox-active but OER-inactive phases on the surface. A LiNiO 2 sample, cycled through the Ni 2+ /Ni III redox, was characterized using operando Raman spectroscopy at 1.56 V (Fig. 4g ). Its Raman spectrum shows clear differences in the position and relative intensity of the Raman bands and a considerable increase in the overall Raman scattering intensity, as compared to pristine LiNiO 2 at the same potential (for more details, see the operando Raman section below). All these spectral features can be indexed to β-NiOOH [50] , indicating the structural transformation of OER-inactive NiOOH species from LiNiO 2 after being cycled through Ni 2+ /Ni III redox. Window-opening voltammetry was also carried out in unpurified 1 M KOH (Supplementary Fig. 19 ), wherein, despite the appearance of the Ni 2+ /Ni III redox peaks in the close potential range, the OER current remains stable even when the lower potential limit reached ~1.11 V. This indicates that Fe impurities significantly improve the performance of NiOOH, in agreement with the common understanding of Ni-based OER electrocatlaysts [38] , [39] , [40] . Therefore, the voltammetric analysis shows that the OER activity and electrochemical properties of LiNiO 2 are impacted by the lower potential limits and presence of Fe impurities in the electrolyte. When undergoing the Ni 2+ /Ni III redox, the surface structure of LiNiO 2 transforms and degrades into NiOOH, which has a poor OER activity in the absence of Fe. In contrast, the pristine and structurally unaltered LiNiO 2 , whose real active species has been covered and neglected in previous LiNiO 2 OER studies [44] , [45] , [47] , [48] , [49] , exhibits better intrinsic OER activity. Operando XRD, XAS, and Raman studies From the aforementioned structural and electrochemical measurements, the pristine nature of LiNiO 2 has been characterised in terms of crystalline phase, local coordination environment, oxidation state and electronic structure, and the superior OER activity of LiNiO 2 to the analogous NiOOH is confirmed and studied in detail. However, the active species of LiNiO 2 , which can no longer be attributed to NiOOH, remains unclear. In addition, LiNiO 2 , a typical cathode material for lithium-ion batteries, can be delithiated to increase the Ni oxidation state and induce structural transition; [24] , [46] therefore, delithiation is expected to become comparable or even easier during the OER in KOH aqueous solution. To establish the relationship between the structure of LiNiO 2 and its OER activity, operando synchrotron-based XRD and XAS, and Raman spectroscopy experiments were carried out. 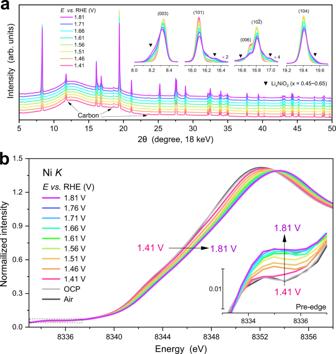Fig. 5: LiNiO2delithiation under OER conditions. aOperando XRD patterns andbOperando NiKedge XANES spectra of LiNiO2under applied potentials of 1.41–1.81 V in 1 M KOH solution. Diffraction peaks in low 2θ ranges and the pre-edge peak were magnified in the corresponding insets. A set of extra peaks are from graphitic carbon and broad diffraction peaks at 12° and 18° from the sample holder. Figure 5a shows the operando synchrotron XRD of LiNiO 2 in 1 M KOH in the potential range of 1.41–1.81 V. The patterns consist of three parts: an amorphous background from cell body and window materials (~12° and 18°), diffraction peaks of graphitic carbon from carbon paper (indicated by arrows), and diffraction patterns of LiNiO 2 and its delithiated derivatives. Using the carbon peak at ~11.8° as the internal reference for intensity and peak position (Supplementary Fig. 20 ), the overall LiNiO 2 pattern largely remains intact under the applied potentials, and another set of pattern emerges with potentials in around 2θ values at the expense of LiNiO 2 pattern intensity when the applied potential is greater than 1.46 V, coinciding with the onset of OER. Whilst (00 l) diffraction peaks of LiNiO 2 show shoulders at lower 2θ values, the (h0l) peaks show shoulders at higher 2θ values, which suggests the formation of another hexagonal phase from the parent LiNiO 2 with interlayer expansion and intralayer contraction for the [NiO 2 ] layers [24] . Based on the peak position, the new phase can be indexed to layered Li x NiO 2 (x = 0.45–0.65, Supplementary Fig. 21 ) [51] , and other Li x NiO 2 polymorphs and NiOOH phases were not found. The LiNiO 2 delithiation during OER is also supported by increased Li concentration of KOH electrolyte and Ni/Li molar ratio of the sample (Supplementary Table 5 ). Considering that both the delithiation and OER initiate from the surface, the delithiated Li x NiO 2 can be considered as the active species of OER. Fig. 5: LiNiO 2 delithiation under OER conditions. a Operando XRD patterns and b Operando Ni K edge XANES spectra of LiNiO 2 under applied potentials of 1.41–1.81 V in 1 M KOH solution. Diffraction peaks in low 2θ ranges and the pre-edge peak were magnified in the corresponding insets. A set of extra peaks are from graphitic carbon and broad diffraction peaks at 12° and 18° from the sample holder. Full size image The oxidation of LiNiO 2 accompanying with delithiation was tracked using operando XANES measurements at the Ni K edge. No discernible change in XANES spectra was observed when the electrode was immersed in 1 M KOH (Supplementary Fig. 22 ). Figure 5b shows the XANES spectra in the potential range of 1.41–1.81 V. The rising edge shifts towards higher energy with the applied potentials, indicating that the oxidation of Ni III coincides with the onset of OER. Using the relationship between the energy at 0.7 edge jump height and the Ni formal oxidation state obtained from ex-situ data (Supplementary Fig. 9 ), the average Ni oxidation state of LiNiO 2 was plotted as a function of the applied potentials (Fig. 6c ). The oxidation state is ~3.0 at 1.41 V, sharply increases to ~3.3 at 1.56 V, gradually at potentials >1.56 V and reaches a plateau of ~3.4. In addition, the pre-edge peak intensity was found to increase with applied potentials (the inset of Fig. 5b ), corresponding to the decreased symmetry of [NiO 6 ] octahedra (see EXAFS analysis below). Combining the potential-dependent oxidation state of Ni with the electrochemistry of LiNiO 2 reveals a positive correlation between the number of Ni IV ions and OER current (Fig. 6c ), suggesting that Ni IV in delithiated Li x NiO 2 can be considered as (part of) the OER active centre. Fig. 6: Local coordination of LiNiO 2 under OER conditions. a , b Fourier transforms of operando Ni K edge EXAFS spectra of LiNiO 2 under applied potentials of 1.41–1.81 V in 1 M KOH solution, with the Ni–O region and the Ni–Ni region magnified to better show the potential-dependent behaviour. The Fourier transformation was carried out over a k range of 2.5 − 12.4 Å −1 , and the Fourier transforms were phase-corrected. c Average oxidation state, N (Ni–O) and R (Ni–O) of LiNiO 2 as a function of applied potentials. The error bars represent the uncertainty of the fitted parameters. d Operando Raman spectra of LiNiO 2 , showing the E g and A 1g vibration bands, where oxygen atoms of [NiO 6 ] units move oppositely along adjacent O-layers and symmetrically along the c-axis, respectively. Full size image The dominance of Ni IV with double ligand hole state (3 d 8 L 2 ) is supported by simulation of the experimental sXAS at the Ni- L 3,2 edge of LiNiO 2 after OER taken with surface sensitive TEY mode (black circles) using the full multiplet cluster calculation which includes full intra-atomic multiplet interaction, crystal field interaction and covalence. We found the experimental Ni- L 3,2 sXAS of LiNiO 2 after OER can be well reproduced by the sum (black line) of 75% 3 d 8 L 2 (blue line) and 25% 3 d 8 L (red line) configurations (Supplementary Fig. 23b ) giving rise to Ni 3.75+ valence state. Potential-dependent changes of LiNiO 2 -raw in XANES are much weaker than those of pure LiNiO 2 (Supplementary Fig. 24 ). The average oxidation state of Ni of LiNiO 2 -raw grows much slower with applied potentials than that of LiNiO 2 , and reaches only ~3.2 at 1.81 V. The impeded Ni oxidation in LiNiO 2 -raw implies that the formation of Ni IV and double ligand hole state in LiNiO 2 -raw is limited. For the LiNiO 2 -raw sample, the XRD patterns show increasing fraction of NiOOH phase with applied potentials, while the R-3m structures is largely maintained in LiNiO 2 without discernible formation of any NiOOH phases (Supplementary Fig. 25 ). It should be noted that the nanoscale thickness of our LiNiO 2 is a prerequisite to observe significant spectral changes in operando XRD and operando XAS, because the OER usually occurs within several nanometres from the surface. Thus, our results indicates that observation of Ni IV with double ligand holes state is directly related to both our pure and nano-sheet pristine LiNiO 2 sample. Potential-dependent changes in the local coordination environment of Ni were probed using operando EXAFS (Fig. 6a, b ). Similar to the ex-situ data, the Ni coordination shell is dominated by Ni–O and Ni–Ni scattering paths. The amplitude of Ni–O at ~1.45 Å increases with the applied potentials from 1.41 to 1.81 V (Fig. 6b ). Because the Ni first-shell coordination in pristine LiNiO 2 is saturated with six oxygen atoms, the coordination numbers (CN) of Ni-O cannot increase further, which alternatively implies the Ni-O bonds become increasingly ordered with the applied potentials. The lowered Ni-O distortion is also suggested by the decreased Ni-O peak border at the high R with increased amplitude (Fig. 6b ) and by the increased frequency of Ni-O oscillation in the real part of the Fourier transforms (Supplementary Fig. 26 ). Quantitative structural information was extracted via EXAFS fitting (Supplementary Fig. 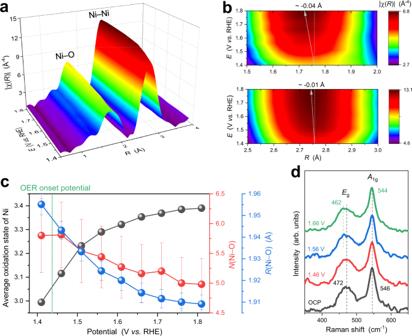Fig. 6: Local coordination of LiNiO2under OER conditions. a,bFourier transforms of operando NiKedge EXAFS spectra of LiNiO2under applied potentials of 1.41–1.81 V in 1 M KOH solution, with the Ni–O region and the Ni–Ni region magnified to better show the potential-dependent behaviour. The Fourier transformation was carried out over a k range of 2.5 − 12.4 Å−1, and the Fourier transforms were phase-corrected.cAverage oxidation state,N(Ni–O) andR(Ni–O) of LiNiO2as a function of applied potentials. The error bars represent the uncertainty of the fitted parameters.dOperando Raman spectra of LiNiO2, showing theEgandA1gvibration bands, where oxygen atoms of [NiO6] units move oppositely along adjacent O-layers and symmetrically along the c-axis, respectively. 27 and Supplementary Table 6 ), where the parameter σ 2 (Ni–O) represents the distortion in the [NiO 6 ] octahedra. The value of σ 2 (Ni–O) decreases as a function of the applied potential from 0.012 Å −2 at 1.41 V to 0.008 Å −2 at 1.81 V, supporting that the LiNiO 2 evolves from the oxidation of SD-active Ni III atoms (t 2g 6 e g 1 ) to SD-inactive Ni IV atoms (t 2g 6 ) under OER. In addition, the CN(Ni–O) decreases from 5.8 ± 0.6 at 1.46 V to 5.0 ± 0.4 at 1.81 V, indicating the formation of oxygen vacancies during OER [52] , [53] , [54] , which have been calculated to greatly reduce the OER overpotential by enhancing intermediate adsorption on the Ni sites [53] , [54] . In addition, the increase in the relative spectral intensity of the weak pre-edge peak at 8335.4 eV in the Ni- K XANES as a function of applied potentials (the inset of Fig. 5b ) implies a reduced local symmetry of Ni ion, which generally suggests a decrease in CN [53] . Moreover, our DEMS measurements and DFT calculation indicate that lattice oxygen involves in OER process (see below). In this lattice oxygen mechanism, oxygen vacancies should be created. In addition to the amplitude, the contour maps of Ni–O shows a gradually increasing contribution in the corresponding lower R regions (Fig. 6b ), corresponding to a shift toward lower R in the real part of FT-EXAFS (Supplementary Fig. 26 ). A shrinking Ni–O bond length from 1.955 Å at 1.41 V to 1.909 Å at 1.81 V was determined via EXAFS fitting (Fig. 6c , Supplementary Fig. 27 and Supplementary Table 6 ), supporting the presence of a high valence state of Ni IV under OER conditions. To summarise, by combining the fast operando Ni- K XANES and EXAFS spectra with the OER onset potential, Ni IV and oxygen vacancies in delithiated Li x NiO 2 were identified during OER, and attributed to the high OER activity. Operando Raman spectroscopy was further employed to track the intermediate species of LiNiO 2 under the high applied potentials larger than 1.4 V. Different from the above Raman experiments in Fig. 4g , the LiNiO 2 now was not forced to undergo Ni 2+ /Ni III redox, but directly applied to 1.46 V. The spectral profile of LiNiO 2 Raman in Fig. 6d only exhibits slightly red-shifted bands ( E g : from 472 cm −1 to 462 cm −1 ; A 1g : from 546 cm −1 to 544 cm −1 ) with increasing applied potentials during the OER process, in agreement with the formation of delithiated LiNiO 2 [55] . This supports the results from the above operando XRD and XAS. From comparison between Fig. 6d and Fig. 4g we can conclude that the crystal structure, intermediates and the OER activity (Fig. 4f ) of LiNiO 2 strongly depend on the lowest potential applied. The presence and formation of γ-NiOOH have been regarded as the origin of OER activity in many Ni-based oxides [46] , [53] , [56] . However, according to our operando Raman spectra (Fig. 6d ), the active species of LiNiO 2 could not be assigned to γ-NiOOH as per the band position and relative intensity (for LiNiO 2 , A 1g : ~546 cm −1 and I( E g )/I( A 1g )=0.5; for γ-NiOOH, A 1g : 558 − 560 cm −1 and I( E g )/I( A 1g ) = 1.5 − 1.7) [40] , [57] , [58] , [59] . In addition, a large expansion in the interlayer spacing between [NiO 2 ] layers, caused by the transformation from LiNiO 2 (4.72 Å) to γ-NiOOH (≥7 Å), was not observed in our operando XRD data. In addition, post-mortem XRD and XAS indicate that the structure of Li x NiO 2 remains mainly intact after OER (Supplementary Fig. 29 and 30 ). Moreover, the surface and bulk AC-STEM images were employed to study the structural transformation of LiNiO 2 after OER [60] , [61] (Supplementary Fig. 31 ), and both show the atomic arrangement perpendicular to the (018) lattice plane of LiNiO 2 , supporting the surface structure of LiNiO 2 remains mainly intact after OER. Thus, using operando X-ray diffraction/absorption and Raman spectroscopies and post-mortem characterizations, the active species were identified as the delithiated yet structurally intact LiNiO 2 with oxygen vacancies. DFT calculation and DEMS for OER mechanisms First-principles DFT calculations were employed to investigate the underlying mechanism of the enhanced OER activity of delithiated LiNiO 2 with respect to the reaction steps. Similar to our previous work [11] , [62] , [63] , three scenarios were considered for the OER mechanisms involving four proton-electron transfer steps: metal-site adsorbate evolution (MAE) mechanism, lattice-oxygen-vacancy-site (LOV) mechanism, and metal-and lattice-oxygen-vacancy-site (MLOV) mechanism. In these mechanisms, the adsorbate sites of the reaction steps are different: only the Ni sites in MAE, oxygen sites in LOV, and both in MLOV (Fig. 7a ). We built models for perfect LiNiO 2 and delithiated Li x NiO 2 to investigate the effects of the unsaturated Ni IV state generated during OER. The (102) plane of LiNiO 2 with a 50% lithium vacancy was used to model the surface reaction pathways on delithiated Li x NiO 2 (x = 0.5, Supplementary Fig. 32 ), as the delithiation and oxidation of LiNiO 2 and the concomitant OER all start from the edge [25] , [52] . Fig. 7: The OER mechanism of LiNiO 2 . a Schematic 4-step reaction pathways of MAE, LOV, and MLOV OER mechanisms. Free energy of each OER step of b Li 0.5 NiO 2 and LiNiO 2 at U RHE = 1.23 V. The estimated thermodynamic overpotentials of each potential-determining step are labelled. c MSCV and faradic CV curves recorded in 18 O-enriched 0.1 M KOH electrolyte prepared using H 2 18 O (99% 18 O), showing the mass ion current ( i MS ) of 18 O 2 , 16 O 18 O and 16 O 2 along with the faradaic current ( i F ) and the applied potential E from the first CV scan. (The inset of c ) Comparison of the measured i MS ( 16 O 18 O) curve and the theoretically expected i MS ( 16 O 18 O) curve purely from electrolyte oxidation, based on the 16 O abundance of 1.18% in the electrolyte (Supplementary Equation S 27 ). d The evolution of measured 18 O abundance of evolved oxygen (from total DEMS charge) for 18 O-labled LiNiO 2 with CV cycles in H 2 16 O-based 0.1 M KOH electrolyte. The expected 18 O fractions are based on the natural isotope abundance and on the measured value from DEMS experiment of unlabelled LiNiO 2 in the 16 O-based electrolyte. Full size image The Gibbs free energy differences (ΔG) of each OER step via the three OER mechanisms for Li 0.5 NiO 2 and LiNiO 2 are shown in Fig. 7b , respectively. First, regardless of the OER pathway, the potential-limiting step of Li 0.5 NiO 2 possess lower overpotential than that of LiNiO 2 , in agreement with the operando measurement results indicating delithiated Li x NiO 2 as the actual active phase for OER. Second, among the three OER scenarios for Li 0.5 NiO 2 the MLOV route shows the lowest overpotential (0.69 V), suggesting that the OER via MLOV prevails on the delithiated Li 0.5 NiO 2 , and that the potential-limiting step is the adsorption of *OH (step 3). Third, for the OER on LiNiO 2 , the MLOV route also prevails, but the potential-limiting step switches to the formation of *OO intermediates and oxygen vacancies (step 1). The transition of the potential-limiting step of LiNiO 2 before and after delithiation can be attributed to the double ligand hole state induced by the presence of Ni IV ions in Li 0.5 NiO 2 . In the electronic structure of octahedral-symmetric [NiO 6 ] system, the charge-transfer energy from the O 2 p to Ni 3 d orbitals decreases with the increased valence state of the Ni ion [4] , [20] , [52] . The LiNiO 2 system is already in the negative charge-transfer regime, and consequently, the Ni-O interaction is highly covalent [14] , [17] , in which Ni III adopts an average configuration close to 3 d 8 L (rather than the formal 3 d 7 ), leaving a ligand hole residing on the O 2 p orbitals. The covalency increases further when the Ni III is (partly) oxidised to Ni IV via LiNiO 2 delithiation, and the resulting Ni IV was endowed with an average configuration of 3 d 8 L 2 , that is, a double ligand hole state in O 2 p . The high unoccupied density state with the O 2 p ligand character in Li x NiO 2 activates lattice oxygen, favouring direct coupling with oxygenated intermediates and the formation of oxygen vacancies (i.e. step 1 of the MLOV route), which are the potential-limiting step of LiNiO 2 . The prediction of oxygen vacancies formation during OER is in good agreement with the experimental observation of operando XAS (Fig. 6c ). Thus, density-functional theory indicates that the double ligand holes created under OER condition easily activates lattice oxygen, accelerating the formation of O-O binding and oxygen vacancies, and the presence of double ligand hole states is closely correlated to the high OER activity of the delithiated Li x NiO 2 . To confirm the participation of lattice oxygen during OER, we performed 18 O-isotope labelling experiments using in situ differential electrochemical mass spectrometry (DEMS). 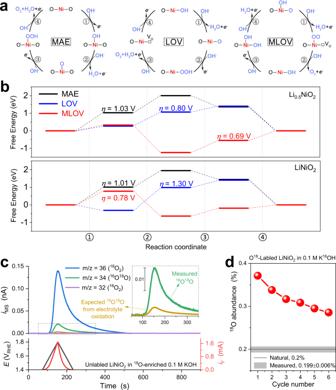Fig. 7: The OER mechanism of LiNiO2. aSchematic 4-step reaction pathways of MAE, LOV, and MLOV OER mechanisms. Free energy of each OER step ofbLi0.5NiO2and LiNiO2at URHE= 1.23 V. The estimated thermodynamic overpotentials of each potential-determining step are labelled.cMSCV and faradic CV curves recorded in18O-enriched 0.1 M KOH electrolyte prepared using H218O (99%18O), showing the mass ion current (iMS) of18O2,16O18O and16O2along with the faradaic current (iF) and the applied potentialEfrom the first CV scan. (The inset ofc) Comparison of the measurediMS(16O18O) curve and the theoretically expectediMS(16O18O) curve purely from electrolyte oxidation, based on the16O abundance of 1.18% in the electrolyte (Supplementary Equation S27).dThe evolution of measured18O abundance of evolved oxygen (from total DEMS charge) for18O-labled LiNiO2with CV cycles in H216O-based 0.1 M KOH electrolyte. The expected18O fractions are based on the natural isotope abundance and on the measured value from DEMS experiment of unlabelled LiNiO2in the16O-based electrolyte. The experiments were first carried out on unlabelled LiNiO 2 in an 18 O-enriched KOH electrolyte (prepared using 99% H 2 18 O) over six consecutive CV cycles from 1.4 V to 1.8 V. Figure 7c shows the first CV and simultaneous mass spectrometric cyclic voltammogram (MSCV) in the time domain. In the MSCV curves, the mass signal m/z = 34 of 16 O 18 O, which is mainly originated from the coupling of 16 O of the LiNiO 2 lattice and 18 O of the electrolyte, shows significant ion current, with 36 O 2 as the dominant molecular oxygen isotope and 32 O 2 within the noise level. The measured 16 O 18 O mass signal was also compared with the theoretically expected profile of the oxidation of the 18 O-enriched electrolyte (1.18% 16 O abundance, the inset of Fig. 7c ), revealing a significant excess of the 16 O 18 O ion charge. This evidences that the lattice oxygen plays a direct role in forming O 2 during OER [4] , [10] , [64] . Furthermore, after the lattice 16 O was partially replaced by 18 O from the electrolyte, the resulting 18 O-labelled LiNiO 2 was cycled in a H 2 16 O-based KOH electrolyte for another six consecutive cycles to study the reverse oxygen isotope replacement (Supplementary Fig. 33 ). The first-cycle data reveal a nearly two-fold 18 O abundance than the expected 18 O fractions from the natural isotope abundance and from the measured value of unlabelled LiNiO 2 in the same O 16 -based electrolyte (Supplementary Fig. 34 and Supplementary Equation S 28 ). The 18 O isotope excess gradually decreases with the number of cycles Fig. 7d ), indicating the consumption of 18 O on the labelled LiNiO 2 in forming O 2 . Therefore, the two-way isotope labelling experiments confirm the participation of LiNiO 2 lattice oxygen in the OER, supporting the predicted MLOV mechanism and activated lattice-oxygen in the presence of double ligand holes. Fe 3+ impurity effects It is widely accepted that the incorporation of Fe 3+ into Ni (oxy)hydroxides promote OER activity by forming synergetic active centres of oxygen-bridged Ni and Fe sites [56] , [65] , and the activity can be further enhanced via structural ordering, as recently proposed by Lee et al. [58] . Structurally intact Li x NiO 2 with stabilised double ligand holes could be a better platform for forming such synergetic centres than the usually amorphous NiOOH. 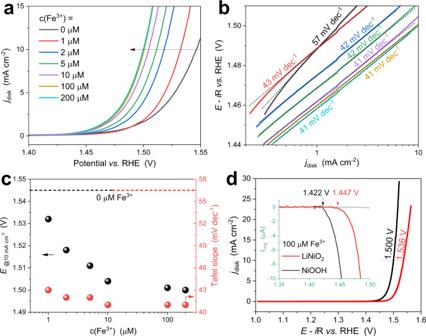Fig. 8: Promotional effects of Fe3+on the OER activity of LiNiO2. aLSVs andbTafel plots of LiNiO2in Fe-free 1 M KOH with the addition of Fe3+solutions (prepared from ultrapure water and Fe(NO3)3∙ 9H2O, 99.999%-Fe, PURATREM, Strem).cPotentials at 10 mA cm−2and Tafel slopes as a function of Fe3+concentrations.dComparison of the Fe3+promotional effects on LiNiO2and NiOOH. Note that 100 µM Fe3+reaches the saturated concentration of Fe(OH)4-(the predominant Fe3+species in alkaline solution)70. Figure 8a compares the linear sweep voltammograms of LiNiO 2 titrated with Fe 3+ in purified 1 M KOH. Similar to the reported Ni (oxy)hydroxides, the OER activity of LiNiO 2 is strongly correlated with the Fe 3+ concentration in terms of E(@10 mA cm −2 ) and Tafel slopes (Fig. 8a–c ): (1) E(@10 mA cm −2 ) decreases with the Fe 3+ concentration and saturated at 1.500 V in the presence of 100 µM Fe 3+ (45 mV lower than that in the Fe-free electrolyte, Figs. 8a ), and (2) the Tafel slope plummets from 57 to 43 mV dec −1 in the presence of only 1 µM Fe 3+ , and largely remains constant up to a Fe 3+ concentration of 200 µM (Fig. 8b ). The decreased Tafel slope at such a low Fe 3+ concentration indicates that OER is switched to a Fe-involving electrocatalytic site with higher activity, and the number of such new active sites increases with Fe 3+ concentration, resulting in Fe-concentration-dependent E(@10 mA cm −2 ). For comparison, NiOOH was also measured in 1 M KOH containing 100 µM Fe 3+ . Although the overall activity is highly promoted as expected (Supplementary Fig. 35 ), NiOOH-Fe 3+ shows 36 mV higher than LiNiO 2 -Fe 3+ in E(@10 mA cm −2 ) and 25 mV in OER onset potential (Fig. 8d ), proving LiNiO 2 an excellent platform for forming Ni-Fe active sites. In addition, the presence of high-valent Ni in Ni-Fe active sites is also found to promote electrocatalytic durability [30] . The promotional mechanism and underlying role of double ligand holes in Ni-Fe lithiated oxide systems are also of interest and related studies are currently underway. Fig. 8: Promotional effects of Fe 3+ on the OER activity of LiNiO 2 . a LSVs and b Tafel plots of LiNiO 2 in Fe-free 1 M KOH with the addition of Fe 3+ solutions (prepared from ultrapure water and Fe(NO 3 ) 3 ∙ 9H 2 O, 99.999%-Fe, PURATREM, Strem). c Potentials at 10 mA cm −2 and Tafel slopes as a function of Fe 3+ concentrations. d Comparison of the Fe 3+ promotional effects on LiNiO 2 and NiOOH. Note that 100 µM Fe 3+ reaches the saturated concentration of Fe(OH) 4 - (the predominant Fe 3+ species in alkaline solution) [70] . Full size image In conclusion, a comprehensive picture correlating electrochemical properties and operando spectroscopies is present to uncover the pristine activity, actual active species, and reaction centres of high-entropy LiNiO 2 for OER. Pristine LiNiO 2 with single-crystalline R-3m structure and with pure Ni III was prepared and characterized unambiguously using electron microscopy, XRD, and XAS. The best and real OER activity of LiNiO 2 is achieved when the electrochemical redox of Ni 2+ /Ni III and the introduction of Fe impurities are prevented, and the activity is found to be comparable with that of the state-of-the-art IrO 2 and much higher than that of the conventional NiOOH in terms of overpotentials, Tafel slopes and OER onset potentials. , Operando XRD, XAS, and Raman spectra were combined to probe the active species and reaction centre. The in situ delithiation, Ni III oxidation and oxygen-vacancy formation in LiNiO 2 under OER were found to coincide with OER for the first time, and the active species was then identified as delithiated yet structurally intact Li x NiO 2 with high-valent Ni IV and double ligand holes, which is also supported by the prevalence of the MLOV OER mechanism from DFT calculation and by the activated lattice oxygen from in situ DEMS measurements. This unique Li x NiO 2 active sites were also found to be superior to those of NiOOH for the formation of a synergetic electrocatalyst with Fe 3+ . This study elucidates the electrocatalysis of lithiated metal oxides in OER and highlights the importance of considerate electrochemical measurements and complementary operando techniques in understanding the pristine electrochemistry and actual active species. Preparation of LiNiO 2 The pristine LiNiO 2 was synthesized using a solid-state reaction method with two annealing steps. NiO and LiOH were grinded and mixed by a mortar and pestle for 30 min, and transferred into a tubular furnace. A 15% excess of the Li precursor was added to compensate for the evaporation of Li 2 O and/or Li 2 O 2 during annealing. After the furnace was purged with O 2 (100 sccm) for 15 min, under such O 2 flow the temperature was increased to 750 °C with a ramping rate of 5 °C min −1 and held at this temperature for 72 h. The second annealing step was carried out at ~100 bar O 2 pressure with cooling naturally to room temperature. Structural characterisation Lab-based X-ray diffraction (XRD) patterns were obtained using a Bruker D8 Advance diffractometer with Cu K α radiation (λ = 1.5418 Å) and a LYNXEYE detector, and diffraction peaks from Cu K α2 was stripped off using Jade 6 software. Transmission electron microscopy (TEM) measurements, including low-magnification TEM, high-resolution TEM (HRTEM) and selected area electron diffraction (SAED), were carried out on a FEI Tecnai G2 F20 S-TWIN electron microscope. Scanning electron microscopy (SEM) measurements were performed on a Zeiss Crossbeam 540. High-angle annular dark-field scanning transmission electron microscopy (HAADF-STEM) images were recorded using an aberration-corrected FEI Themis Z STEM. The microscope was operated with an accelerating voltage of 60 kV and the HAADF detector angle range was 50–200 mrad. Note that the accelerating voltage of STEM was selected as 60 kV to prevent beam damage, which is reported to induce Ni displacement and oxygen release on LiNiO 2 after long exposure to electron irradiation [66] . X-ray absorption spectra (XAS) at the Ni K edge were measured in the transmission mode at TPS 44 A beamline of National Synchrotron Radiation Research Centre (NSRRC, Hsinchu), and using an in-house lab-based X-ray absorption spectrometer (Supplementary Fig. 36 ). The electron storage ring of the TPS was operated at 3.0 GeV with a ring current of ~500 mA. The measured spectra were processed and analysed using ATHENA and ARTEMIS (Demeter software package) [67] . Soft XAS (sXAS) at the Ni L 3,2 edge and the O K edge were collected at TLS 11 A and 20 A beamlines of the NSRRC. The Ni L edge data of γ-NiOOH and KNiIO 6 were measured in fluorescence mode and inverse partial fluorescence yield mode, respectively, to reduce the spectral distortion of surface Ni 2+ . Electrochemical measurements Electrochemical measurements were performed on a standard three-electrode setup connected to a PGSTAT302N potentiostat (Metrohm Autolab, equipped with FRA32M and BA modules). A Pt gauze was used as the counter electrode, and a Hg|HgO electrode (in 1 M KOH) as the reference electrode. The potential measured using the Hg|HgO reference electrode, E(V vs. Hg|HgO, 1 M KOH), was converted into RHE scale in 1 M KOH, E(V vs. RHE), using the following equation, E(V vs. RHE) = E(V vs. Hg|HgO, 1 M KOH) + 0.0977 V + 0.05916 pH (V) (1) , where the pH of the purified 1 M KOH is measured as 13.73 at 25 °C. The values of potential in the text are thus referenced against RHE, unless stated otherwise. The contact and solution resistance were determined using electrochemical impedance spectroscopy under open circuit potential (OCP) before each voltammetry measurement, and the voltammograms were corrected by IR drops. The working electrode was prepared by drop-casting 10 μL of a catalyst ink onto a polished rotating ring-disk electrode (RRDE, with a glassy carbon disk and a Pt ring) and drying under ambient condition to obtain an even film. The catalyst ink was prepared by dispersing 5 mg of each sample and 5 mg carbon (Vulcan XC-72R) into 1 mL isopropanol alcohol (IPA) aqueous solution (25 vol% of IPA) containing 40 μL 5 wt% Nafion solution. Linear sweep voltammograms and cyclic voltammograms (CV) were collected using a RRDE configuration with 5 mV s −1 in Ar-saturated 1 M purified KOH solution at 25 °C. The voltammograms were collected at 1600 rpm to promptly remove the generated O 2 , and the disk potential was swept from the corresponding OCP of each sample, while the ring potential was held at −0.5 V (vs. Hg|HgO, 1 M KOH) to electrochemically reduce and detect the O 2 evolved from the disk. For the long-term stability test, the working electrode was prepared using carbon paper (Toray TGP-H-060) with the same catalyst loading and ink recipe as the RRDE, and the stability was evaluated using chronopotentiometry at 10 mA cm −2 for 48 h, before and after which LSV curves were measured with 5 mV s −1 . The OER activity of NiOOH and IrO 2 (99.9%, Adamas-beta) was measured for comparison. The NiOOH was prepared by potential cycling NiO nanopowder (50 nm, 99.9% metal basis, Aladdin) in 1 M KOH between 1.01 V and 1.66 V for at least 40 cycles until the Ni 2+ /Ni III redox couple at ~1.32 V was fully developed (Supplementary Fig. 37 ). To avoid the inference of Fe impurities on the measured OER activity, the electrochemical cell was cleaned by concentrated H 2 SO 4 overnight and boiled with ultrapure H 2 O (18.2 MΩ cm) for at least 3 times to remove residual H 2 SO 4 and other impurities, and the KOH solution was purified using Trotochaud’s method [38] . Briefly, 1 M KOH solution was first prepared from semiconductor grade KOH (99.9996% metal basis, 4 ppm total metal impurity excluding Na + , Aladdin) and ultrapure water. Into a H 2 SO 4 -rinsed 50 mL polypropylene centrifuge tube, ~2 g of Ni(NO 3 ) 2 ·6H 2 O (99.9985%, PURATREM, STREM) were dissolved in ~4 mL ultrapure H 2 O and mixed with 20 mL 1 M KOH. The resulting Ni(OH) 2 suspension was shaken and centrifuged, and the supernatant was decanted. The Ni(OH) 2 was then washed 3 times with ~20 mL ultrapure H 2 O and ~2 mL 1 M KOH, and transferred to a H 2 SO 4 -rinsed 100 mL polypropylene bottle. The bottle was filled with 75 mL 1 M KOH for purification, and the freshly prepared and washed Ni(OH) 2 was redispersed and shaken for 10 min, followed by resting overnight. Operando and online characterisation Operando synchrotron XRD patterns were collected at TLS 01C2 beamlines of the NSRRC. The XRD experiments were performed at an incident beam energy of 18 keV using a mar345 image plate area detector. The diffraction intensity and the peak shape were calibrated with a CeO 2 reference sample (SRM 674b). Operando Quick - XAS measurements at Ni K were carried out in the transmission mode at TPS 44 A beamline of the NSRRC, and 120 XAS spectra collected within 1 min were merged to achieve high data quality. Operando Raman spectra were collected using a Horiba LabRAM HR Evolution confocal Raman microscope with an excitation wavelength of 473 nm. The spectra resolution is ~1 cm −1 , and the spectral shifts were calibrated routinely using silicon wafer (520.7 cm −1 ). The operando Raman experiments were performed in a homemade spectro-electrochemistry cell, consisting of a Au disk working electrode (5 mm), a Pt wire counter electrode and a Ag|AgCl (saturated KCl) reference electrode. Online differential electrochemical mass spectrometry (DEMS) measurements were carried out using a QAS-100 equipped with a PrismaPro quadrupole mass spectrometer (Linglu Instruments). The O 18 -labeled LiNiO 2 was prepared by cycling the unlabelled one to the OER range (e.g., 1.8 V) in 18 O-enriched electrolyte, and before the experiment in the 16 O-based electrolyte, rinsing and drying steps were conducted to remove free 18 O species. Computation details The present calculations employ the Vienna ab initio Simulation Package (VASP) implementation of density functional theory (DFT) in conjunction with the projector augmented wave (PAW) formalism [68] . The H 1 s 1 , Li 2 s 1 , O 2 s 2 2 p 4 , and Ni 4 s 2 3 d 8 states are treated as valence electrons. The electronic wave functions were expanded in plane waves using an energy cutoff of 520 eV, and the force and energy convergence criteria were set to 0.02 eV Å −1 and 10 −5 eV respectively. To overcome the self-interaction error of the exchange correlation functional, we employed the Hubbard U model for describing the strong correlation of the localized Ni 3 d states, and set the value of U eff = ( U − J) to 6.40 eV according to previous work [46] . The reciprocal space was sampled using a 4×4×1 Monkhorst–Pack k -point mesh for DFT + U calculations. To simulate the valence states of Ni in real catalytic environment, we built the Li 0.5 NiO 2 system containing 50% lithium vacancy. The periodic slab models of LiNiO 2 and Li 0.5 NiO 2 system with 9 Ni sites per surface, with two layers at the bottom fixed during the relaxation. To prevent spurious interactions, the thickness of vacuum spacing was ~15 Å in the z-direction . We calculated the Gibbs free-energy differences (∆G) using the computational hydrogen electrode model under standard conditions [69] , with the voltage applied U RHE = 0 and 1.23 V. The calculation details regarding ∆G can be found in the Supplementary Information.